Wavefront modulation and subwavelength diffractive acoustics with an acoustic metasurface Metasurfaces are a family of novel wavefront-shaping devices with planar profile and subwavelength thickness. Acoustic metasurfaces with ultralow profile yet extraordinary wave manipulating properties would be highly desirable for improving the performance of many acoustic wave-based applications. However, designing acoustic metasurfaces with similar functionality to their electromagnetic counterparts remains challenging with traditional metamaterial design approaches. Here we present a design and realization of an acoustic metasurface based on tapered labyrinthine metamaterials. The demonstrated metasurface can not only steer an acoustic beam as expected from the generalized Snell’s law, but also exhibits various unique properties such as conversion from propagating wave to surface mode, extraordinary beam-steering and apparent negative refraction through higher-order diffraction. Such designer acoustic metasurfaces provide a new design methodology for acoustic signal modulation devices and may be useful for applications such as acoustic imaging, beam steering, ultrasound lens design and acoustic surface wave-based applications. Recent years have witnessed the emergence of a family of planar wave modulation devices, known as metasurfaces [1] , [2] , [3] , [4] , [5] , [6] . These engineered surfaces of subwavelength thicknesses are capable of many forms of wave manipulation and thus have drawn significant attention from both physics and engineering communities. Not only do these metasurfaces inspire the revisiting of fundamental physical laws governing wave propagation, but also they promise a bright future for useful devices with extremely compact footprint. Electromagnetic metasurfaces have been experimentally realized with optical antennas or microwave metamaterials [1] , [2] , [3] , [4] , [5] , [6] . However, mapping the success of electromagnetic metasurfaces to the acoustic domain is challenging, mostly due to the mechanical nature and distinct properties of acoustic waves. Some initial theoretical exploration [7] , [8] has recently been shown, nevertheless, only limited experimental investigations have been demonstrated [9] . In this work, we demonstrate an acoustic metasurface capable of general wavefront modulation through four distinct wave manipulation properties: anomalous refraction, conversion from propagating wave to surface evanescent mode, extraordinary beam-steering and apparent negative refraction through higher-order diffraction. We verify that the generalized Snell’s law provides an accurate description for the first two properties. The last two properties, in contrast, are produced from the interaction of the periodicity of the metasurface and the spatially varying phase modulation, creating an additional term in the generalized Snell’s law. Our metasurface is essentially a metamaterial/phononic crystal hybrid structure [10] and both the local and non-local responses can be leveraged for the purpose of shaping the wavefront with a much larger degree of control than traditional acoustic wave manipulation methods. Such thin planar acoustic metasurfaces, along with existing bulk metamaterials [11] , [12] , [13] , [14] , [15] , [16] , [17] , [18] , [19] , [20] , provide a new design methodology for acoustic wave modulation, sensing and imaging applications. Engineering surface phase gradient and anomalous refraction To design a metasurface with subwavelength thickness, planar profile and nearly arbitrary wavefront modulation, demanding requirements need to be placed on the material parameters. A recently proposed category of acoustic metamaterials, termed labyrinthine metamaterials [14] , [21] , [22] , shows promise as building blocks for such wavefront-shaping metasurfaces. This family of unit cells features high energy throughput, broad complex (amplitude and phase) modulation range and non-resonant dispersion. Under the guidance of the generalized Snell’s law [1] , we therefore designed our metasurface based on a series of tapered labyrinthine metamaterials [22] . ( Fig. 1a is a concept schematic of our planar acoustic metasurface and the generalized Snell’s law. Also see Supplementary Fig. 1 for the geometry and dimensions of the designed unit cells). The classical Snell’s law rests on the assumption that the accumulated phase is continuous across the interface. 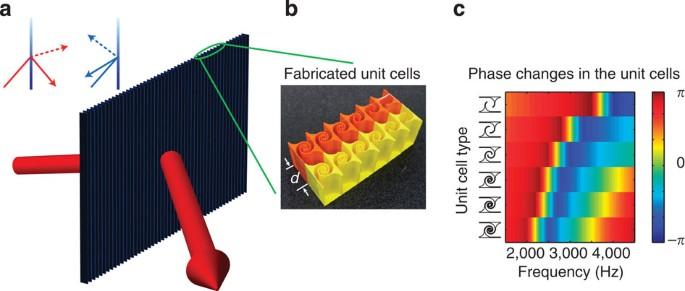Figure 1: Wavefront modulating thin planar metasurface and its constituting elements. (a) Concept schematic of a planar acoustic metasurface and the generalized Snell’s law. Dashed arrow line indicates the positive refraction/reflection ray (corresponding to the modulation effect described by the generalized Snell’s law) and solid arrow line indicates the negative refraction/reflection ray (corresponding to the hybrid response with the contribution from both the local and non-local effects). (b) Photograph of the fabricated unit cell prototypes. (c) Six types of unit cells and the corresponding phase changes through the unit cells. However, introduction of abrupt phase variation generalizes Snell’s law with an extra term describing the phase gradient on the surface : Figure 1: Wavefront modulating thin planar metasurface and its constituting elements. ( a ) Concept schematic of a planar acoustic metasurface and the generalized Snell’s law. Dashed arrow line indicates the positive refraction/reflection ray (corresponding to the modulation effect described by the generalized Snell’s law) and solid arrow line indicates the negative refraction/reflection ray (corresponding to the hybrid response with the contribution from both the local and non-local effects). ( b ) Photograph of the fabricated unit cell prototypes. ( c ) Six types of unit cells and the corresponding phase changes through the unit cells. Full size image By engineering the phase gradient term, nearly arbitrary wavefront modulation can be realized—including focusing, beam steering, conversion from cylindrical wave to plane wave to name a few. Figure 1b,c showcase six types of tapered labyrinthine unit cells [23] with different complex modulation. This set of unit cells have uniform thickness ( d in Fig. 1b ) that is around 25–35% of the wavelength of the interested frequency range (2,500–3,500 Hz) and the difference of their modulated phase change can cover a complete 2 π range with single layer (reflective case) or double layers (transmissive case). Fig. 1c plots the phase change in each type of unit cell over the interested frequency range. At 3,000 Hz, the difference of phase change between adjacent types of unit cell is about π /6 and the phase difference is roughly preserved over a broad bandwidth. (This broadband effect is shown in Supplementary Fig. 2 ). A transmissive metasurface composed of this set of unit cells approximates a phase gradient of 2 π / γ , where γ is the array period of the metasurface (we define the array period as the width of six unit cells. The dimension is shown in Supplementary Fig.1 ). The generalized Snell’s law predicts the transmitted angle to be , although as we show below, an additional term can be important due to the periodicity of the six unit cell array. We first examine the case of normal incidence, that is, θ i =0. Here two metasurfaces with different gradient of phase ξ were investigated using the experimental setup shown in Fig. 2a . The measurement results for ξ =0, , were compared with the theoretical transmitted angles calculated with the generalized Snell’s law (shown as the blue solid curve in Fig. 2b ) and excellent agreement is found. The field patterns corresponding to these three different phase gradients are shown in Fig. 2c . The physics of oblique incidence is much richer and will be explored in the subsequent parts of this paper. 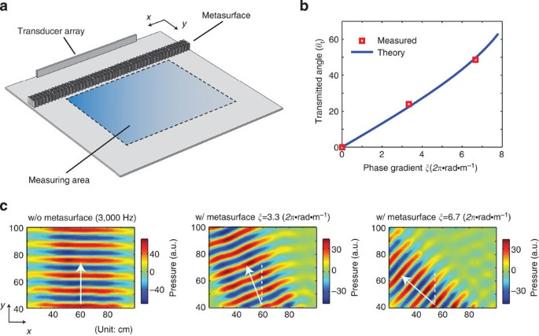Figure 2: Anomalous refraction measurements. (a) Experimental setup. The top plate of the waveguide (not shown in the diagram) is located 50.8 mm above the bottom plate. Blue region is the measuring area and the starting line of the measuring zone (y=40 cm) is 3.4 cm away from the exiting interface of the metasurface. (b) Relation between the transmitted angles and the phase gradients of the metasurfaces at normal incidence. Blue solid line is the theoretical prediction fromand red squares are the measured values. The corresponding measured field patterns for these three phase gradients are shown inc. Figure 2: Anomalous refraction measurements. ( a ) Experimental setup. The top plate of the waveguide (not shown in the diagram) is located 50.8 mm above the bottom plate. Blue region is the measuring area and the starting line of the measuring zone ( y =40 cm) is 3.4 cm away from the exiting interface of the metasurface. ( b ) Relation between the transmitted angles and the phase gradients of the metasurfaces at normal incidence. Blue solid line is the theoretical prediction from and red squares are the measured values. The corresponding measured field patterns for these three phase gradients are shown in c . Full size image Evanescent surface mode converted from propagating wave When the incident angle θ i approaches a certain critical angle θ c , the transmitted wave will bend towards the surface and then become evanescent on the transmitted side. A theoretical estimate using a simple model with continuously varying phase modulation gives the value of the critical angle as for the case of . The measured field pattern for θ i =25° (this angle is located around the centre of the blue region) is shown in Fig. 3a where the non-radiating surface mode can be clearly seen. Fig. 3b shows the spatial Fourier transform of the measured near-field along the surface, which proves that the modulated wave has a transverse wave vector larger than that of the free-space propagation and thus the wave vector component perpendicular to the surface has an imaginary value . The surface mode created is a so-called ‘driven’ surface wave described by Sun et al. [3] and is used as an efficient way to convert propagating waves in free space to surface waves. ‘Driven’ surface wave is different from propagating surface waves in that the field remains localized to the incident field region. According to simulations, when the system is lossless, converted energy will re-radiate back towards the incident side (see Supplementary Fig. 3 ). However, when the system has a small but realistic amount of loss, the reflected energy is significantly reduced (see Supplementary Fig. 4 ). Fig. 3c compares the scattered field patterns between the cases of θ i =20° (within the surface mode region) and θ i =10° (in the transmitting region). Only 27.8% of the incident energy is scattered in the former case while 89.0% is scattered for the latter. In the absence of a means for escape, the majority of the incident energy is absorbed for the case of the evanescent transmission. However, if a proper coupling mechanism is provided, the ‘driven’ surface mode can be efficiently coupled to a propagating surface wave structure. (See Supplementary Note 1 and Supplementary Fig. 5 for more results and discussions). 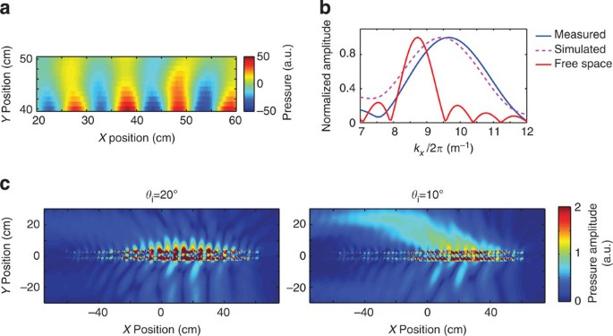Figure 3: Measured and simulated results of the evanescent surface mode. (a) Measured near-field of the evanescent mode on the transmitted side forθi=25°. (b) Spatial Fourier transform of the measured near-field pressure along the metasurface, compared with the simulated result and reference free-space wave vector to prove the evanescent nature of the generated mode. (c) Scattered fields obtained from simulation forθi=20° andθi=10°. Figure 3: Measured and simulated results of the evanescent surface mode. ( a ) Measured near-field of the evanescent mode on the transmitted side for θ i =25°. ( b ) Spatial Fourier transform of the measured near-field pressure along the metasurface, compared with the simulated result and reference free-space wave vector to prove the evanescent nature of the generated mode. ( c ) Scattered fields obtained from simulation for θ i =20° and θ i =10°. Full size image Extraordinary beam-steering and apparent negative refraction When the array period is comparable with wavelength, non-local effects from periodicity will play a crucial role in wave propagation, and the generalized Snell’s law of refraction/reflection will become wave-vector dependent. Under this condition, equation (1) can be reformulated as where G is the amplitude of the reciprocal lattice vector. The structure can be regarded as a phononic crystal whose lattice element is a set of inhomogeneous and dispersive metamaterial unit cells [10] . In one-dimensional case, isofrequency surface analysis can be used for predicting the diffractive properties of the incident wave. 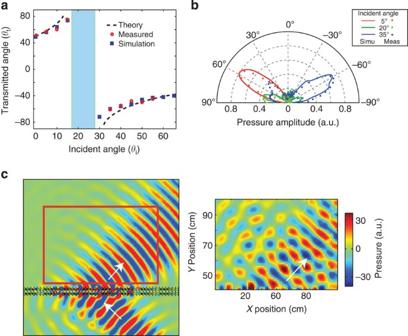Figure 4: Extraordinary beam-steering and negative refraction. (a) Relation between incidence angleθiand transmitted angleθt. The theoretical curve is calculated based on the generalized Snell’s law with the non-local termnGGtaken into consideration (equation (2)). (b) Polar plot of the measured (dots) and simulated (solid lines) radiation patterns for incident angle of 5° (<θc), 35° (>θc) and 20° (aroundθc). (c) Field pattern at 45° (left: simulation, right: measurement), demonstrating the negatively refracted transmission whenθi>θc. The white arrows indicate the forward phase propagation directions. Figure 4a plots the measured θ t versus θ i data and compares it with the simulated data, as well as the theoretical predication. The theoretical curve is calculated from equation (2) where a non-local term n G G is integrated into the generalized Snell’s law. For an incident angle smaller than the critical angle θ c , it can be proven with classical diffraction theory that n G =0. However, when θ i > θ c (the right side of the blue region in Fig. 4a ), n G will jump to a non-zero value ( n G =−3 for our design) as required by the surface momentum matching condition. (a more detailed analysis can be found in Supplementary Note 2 ). Therefore, the θ t versus θ i curve exhibits an abrupt change when θ i crosses the non-radiating region and a very small perturbation of the input signal θ i will lead to a significant shift in the output signal θ t . This phenomenon is related to the passing off orders found in diffractive grating anomalies [23] , [24] . Fig. 4b plots the simulated and measured transmitted field patterns for incident angle of 5°, 20° and 35°. The measured data are normalized with the maximum amplitude of the corresponding simulated data to aid comparison and good agreement is obtained. (A small side lobe for the 35° incidence case might be due to the fabrication defect of the sample.) Such extraordinary beam-steering effect is different from those beam forming or redirecting methods based on active transducer array [25] , [26] or passive materials [27] (including metamaterials [28] , [29] ). Potential applications include acoustic switching and surface wave sensing [30] . It is also worth noting that in the non-local regime (the right side of the blue region in Fig. 4a ), the transmitted beam exhibits negative refraction (refracted beam is on the same side of the incident beam with respect to the surface normal, the field pattern for incident angle of 45° is shown as an example in Fig. 4c ). This is different from the traditional negative refraction phenomena that are usually obtained with bulk negative refractive index metamaterials or phononic crystals; our metasurface achieves the same effect with the modulation from the subwavelength thin interface. Figure 4: Extraordinary beam-steering and negative refraction. ( a ) Relation between incidence angle θ i and transmitted angle θ t . The theoretical curve is calculated based on the generalized Snell’s law with the non-local term n G G taken into consideration (equation (2)). ( b ) Polar plot of the measured (dots) and simulated (solid lines) radiation patterns for incident angle of 5° (< θ c ), 35° (> θ c ) and 20° (around θ c ). ( c ) Field pattern at 45° (left: simulation, right: measurement), demonstrating the negatively refracted transmission when θ i > θ c . The white arrows indicate the forward phase propagation directions. Full size image In conclusion, we have designed and demonstrated an acoustic metasurface that produces arbitrary complex modulations of an incident wavefront. On the basis of tapered labyrinthine unit cells, the metasurface is shown to efficiently redirect incident acoustic beams as described by the generalized Snell’s law. We also demonstrate that, when illuminated beyond the critical angle, the metasurface can convert the incident propagating wave to evanescent surface mode. Last, we demonstrate a regime where periodicity of the metasurface also influences the transmitted energy, creating effects such as extraordinary beam-steering and apparent negative refraction through higher-order diffraction. Our work opens the door to the arena of subwavelength diffractive acoustic devices that can be designed to achieve nearly arbitrary complex modulation of the wavefront. With these ultralow profile planar acoustic metasurfaces, we can expect novel acoustic signal modulation, sensing and imaging applications in the near future. Field mapping measurement The unit cells were made of acrylonitrile butadiene styrene thermal plastics and were fabricated using the fused filament fabrication three-dimensional printing technology. The field mapping measurement was performed in our lab-made two-dimensional acoustic waveguide [31] , [32] . A linear transducer array was used to generate a plane wave with a Gaussian amplitude profile along the wave front and a microphone was swept over the measuring area by a two-dimensional linear stage to record the transmitted wavefronts. Detailed experimental setup and method of measurement can be found in Supplementary Fig. 6 . Numerical simulations The simulation was performed with the commercial finite element analysis solver COMSOL Multiphysics. The unit cell design was based on a standard effective acoustic parameter retrieval method [33] . The pressure field pattern simulation was performed by approximating the experimental conditions of the two-dimensional waveguide measurement system. The boundaries of the calculating area were set to plane wave radiation boundary condition. How to cite this article: Xie, Y. et al. Wavefront modulation and subwavelength diffractive acoustics with an acoustic metasurface. Nat. Commun. 5:5553 doi: 10.1038/ncomms6553 (2014).